TSC1 controls macrophage polarization to prevent inflammatory disease Macrophages acquire distinct phenotypes during tissue stress and inflammatory responses, but the mechanisms that regulate the macrophage polarization are poorly defined. Here we show that tuberous sclerosis complex 1 (TSC1) is a critical regulator of M1 and M2 phenotypes of macrophages. Mice with myeloid-specific deletion of TSC1 exhibit enhanced M1 response and spontaneously develop M1-related inflammatory disorders. However, TSC1-deficient mice are highly resistant to M2-polarized allergic asthma. Inhibition of the mammalian target of rapamycin (mTOR) fails to reverse the hypersensitive M1 response of TSC1-deficient macrophages, but efficiently rescues the defective M2 polarization. Deletion of mTOR also fails to reverse the enhanced inflammatory response of TSC1-deficient macrophages. Molecular studies indicate that TSC1 inhibits M1 polarization by suppressing the Ras GTPase–Raf1–MEK–ERK pathway in mTOR-independent manner, whereas TSC1 promotes M2 properties by mTOR-dependent CCAAT/enhancer-binding protein-β pathways. Overall, these findings define a key role for TSC1 in orchestrating macrophage polarization via mTOR-dependent and independent pathways. Macrophages play an essential role in tissue homeostasis; they orchestrate the initiation and resolution phases of both innate and adaptive immunity, with significant impact on protective immunity and immune-mediated pathological damage [1] , [2] . It is generally believed that macrophages represent a spectrum of activated phenotypes rather than stable subpopulations. Traditionally, macrophages can be polarized into two distinct phenotypes, that is, the classically activated macrophages (M1) and alternatively activated macrophages (M2) (ref. 3 ). M1 macrophages, which are generally considered to be potent effector cells in response to microbial products or interferon-γ (IFN-γ), are characterized by high antigen-presenting capacity, production of proinflammatory cytokines such as interleukin-12 (IL-12) and tumour necrosis factors (TNF-α), nitric oxide (NO) and reactive oxygen intermediates, and consequently, promote a polarized type I immune response to mediate host defence against infections of bacteria, protozoa and viruses as well as tumour cells. In contrast, M2 macrophages, which are induced by IL-4, IL-13, glucocorticoids, IL-10 and immunoglobulin complexes/Toll-like receptor ligands, display anti-inflammatory function, promote adaptive Th2 immunity and regulate angiogenesis, tissue remodelling and wound healing. The balance of M1 and M2 macrophages and the appropriate resolution of macrophage inflammatory response are critical for host homeostasis. The importance of innate immune response in triggering autoimmune diseases has been recognized in mouse models [4] , [5] , [6] . Although it is well recognized that the transcriptional response triggered by surrounding microenvironments, including cytokines, growth factors and microorganism-associated molecular patterns, shapes the phenotype and function of macrophages [7] , [8] , [9] , the intrinsic molecular mechanisms steering macrophage polarization have not been fully elucidated. Mutations in tuberous sclerosis complex 1 (TSC1) or TSC2 give rise to the hamartoma syndrome and the proliferative lung disorder lymphangioleiomyomatosis [10] . TSC1 and TSC2 proteins form a heterodimeric complex that acts as a functional unit and are closely involved in a wide range of cellular functions [10] , [11] , [12] , [13] . TSC1 enhances TSC2 activity by stabilizing TSC2 (ref. 14 ). Studies have shown that TSC2 is the catalytic GTPase-activating protein (GAP) and directly inhibits Rheb small GTPase upstream of mTORC1 complex, so as to downregulate mTORC1 activity [15] , [16] , [17] , [18] . In contrast, TSC1/2 complex is essential for mTORC2 complex activation, which phosphorylates AKT on Ser473 (refs 19 , 20 ). Under certain conditions, TSC2 is phosphorylated and inactivated by the protein kinase AKT, which itself is activated by the phosphatidylinositol 3-kinase (PI3K) pathway [16] , [21] . Current reports on the involvement of TSC1/2-mammalian target of rapamycin (mTOR) in the regulation of innate inflammation are contradictory and limited. The mTOR-specific inhibitor rapamycin (Rapa) showed diverse effects on the functions of dendritic cells (DCs) [22] , [23] , [24] , [25] , [26] . Rapa enhanced IL-23 and other inflammatory cytokine production in macrophages via enhancing nuclear factor κB (NF-κB) and blocking STAT3 activity [27] , [28] . Rapa significantly blocked the anti-inflammatory effects of glucocorticoids in myeloid immune cells including monocytes and DCs [29] . Rapa treatment enriched NF-κB-related proinflammatory cytokines expression and monocyte lineage-specific transcripts in kidney-transplanted recipients [30] . TSC2 −/− mouse embryonic fibroblasts or TSC2-knockdown human acute monocytic leukaemia cell line (THP1) expressed less IL-12 and TNF-α but more IL-10 (ref. 28 ). In contrast, it was reported that TSC1 negatively regulates M1 macrophage function by controlling mTORC1 and JNK1/2 activation [31] . Recently, studies by Horng’s group nicely showed that TSC1KO macrophages are refractory to IL-4-induced M2 polarization, but produce increased inflammatory responses to proinflammatory stimuli [32] . In the present study, we use mice with a myeloid cell-specific deletion of TSC1 gene to investigate the role of TSC1 pathways in the regulation of innate immunity. We herein confirm that macrophages in these mice are skewed towards M1 response while M2 reaction is blocked both in vivo and in vitro . Molecular and biochemical mechanism studies indicate that the enhanced M1 response in TSC1KO mice is mTOR-independent but rather relies on the activation of the Ras GTPase–Raf1–MEK1/2–extracellular signal-regulated kinase (ERK) pathway. But inhibition of M2 response by TSC1 deficiency is mediated through an mTOR-dependent CCAAT/enhancer-binding protein-β (C/EBPβ) pathway. Our results, therefore, indicate that TSC1 plays a critical role in the balance of macrophage polarization via both mTOR-dependent and independent pathways. TSC1/2 expression in polarized macrophages The expression patterns of TSC1 and TSC2 in macrophages with lipopolysaccharide (LPS) and IL-4 stimulation, respectively were determined using real-time PCR and western blots. As shown in Fig. 1 , TSC1 and TSC2 were expressed in primary mouse peritoneal macrophages regardless of LPS and IL-4 stimulation. However, LPS failed to alter TSC1 and TSC2 messenger RNA (mRNA) and protein expression within 48 h as determined by real-time PCR and western blots ( Fig. 1a–c ). But IL-4 significantly increased TSC1 mRNA expression in macrophages ( P <0.01, Fig. 1a ). At the protein level, TSC1 and TSC2 expression was increased only after IL-4 treatment ( Fig. 1d ). It is known that TSC2 activity is downregulated by phosphorylation [16] . Importantly, the phosphorylation of TSC2 including p-TSC2 (939) and p-TSC2 (1462) increased after macrophages were treated with LPS and IL-4, respectively ( Fig. 1c,d ). Consistent with the notion that TSC1/2 complex is a critical negative regulator of mTOR [20] , the downregulation of TSC2 function by phosphorylation led to an increased mTOR activity after LPS and IL-4 stimulation as indicated by the increased p-S6 levels ( Fig. 1c,d ). We thus had a working hypothesis that TSC1/2 complex might be involved in the regulation of macrophage polarization. 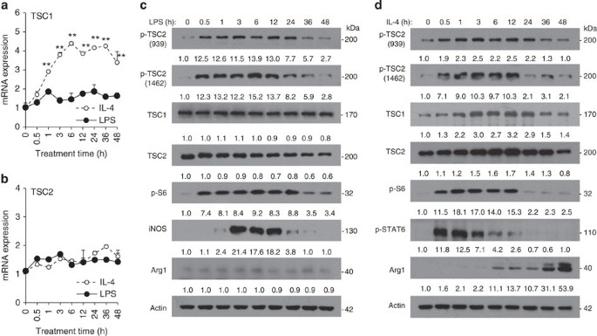Figure 1: TSC1/2 expression and activity are regulated during macrophage polarization. (a) Primary macrophages freshly isolated from the peritoneal cavity of C57BL/6 mice were stimulated with either LPS (100 ng ml−1) or IL-4 at indicated time points. The TSC1 mRNA expression was determined by real-time PCR. (b) TSC2 mRNA expression in primary macrophages was determined by real-time PCR after LPS or IL-4 stimulation. Data are shown as mean±s.d. (N=4), representing one of three independent experiments. **P<0.01 compared with control group. Data were analysed by two-way ANOVA analysis using SPSS software. (c) The levels of p-TSC2(939), p-TSC2(1462), p-S6, TSC1, TSC2, iNOS, Arg and Actin in LPS-stimulated macrophages were determined by western blots. (d) The levels of p-TSC2(939), p-TSC2(1462), p-S6, TSC1, TSC2, p-STAT6, Arg1 and Actin in IL-4-stimulated macrophages were determined by western blots. Images have been cropped for presentation; full-size blot is shown inSupplementary Fig. 23. The relative OD values of each band to LPS-untreated control sample were shown under each band. One of the three independent experiments with identical results was shown. Figure 1: TSC1/2 expression and activity are regulated during macrophage polarization. ( a ) Primary macrophages freshly isolated from the peritoneal cavity of C57BL/6 mice were stimulated with either LPS (100 ng ml −1 ) or IL-4 at indicated time points. The TSC1 mRNA expression was determined by real-time PCR. ( b ) TSC2 mRNA expression in primary macrophages was determined by real-time PCR after LPS or IL-4 stimulation. Data are shown as mean±s.d. ( N =4), representing one of three independent experiments. ** P <0.01 compared with control group. Data were analysed by two-way ANOVA analysis using SPSS software. ( c ) The levels of p-TSC2(939), p-TSC2(1462), p-S6, TSC1, TSC2, iNOS, Arg and Actin in LPS-stimulated macrophages were determined by western blots. ( d ) The levels of p-TSC2(939), p-TSC2(1462), p-S6, TSC1, TSC2, p-STAT6, Arg1 and Actin in IL-4-stimulated macrophages were determined by western blots. Images have been cropped for presentation; full-size blot is shown in Supplementary Fig. 23 . The relative OD values of each band to LPS-untreated control sample were shown under each band. One of the three independent experiments with identical results was shown. Full size image TSC1 controls M1 polarization in an mTOR-independent fashion To address the role of TSC1 in macrophage polarization, we generated mice with TSC1 deletion, specifically in myeloid cells by crossing TSC1 loxp/loxp mice with transgenic mice that carried lysozyme (LysM) proximal promoter-mediated Cre recombinase, in which the target gene was specifically ablated from macrophages and neutrophils as previously reported [33] . After several rounds of crossing, we obtained mice with TSC1 homozygous deletion in myeloid cells ( LysMCreTSC1 loxp/loxp ; herein referred to as TSC1KO), and wild-type (WT) mice ( TSC1 loxp/loxp ). Selective deletion of TSC1 exons 17 and 18 by LysMCre-mediated recombination in peripheral monocytes/macrophages, partially in granulocytes, but not in T cells and B cells was determined by real-time PCR and western blot assays ( Supplementary Fig. 1 ). The TSC1KO macrophages expressed normal levels of CD14 and TLR4 molecules as did WT macrophages ( Supplementary Fig. 2 ), indicating that the TSC1/2 complex does not directly regulate CD14 and TLR4 expression on macrophages. However, LPS or LPS plus IFN-γ treatment induced significantly more TNF-α, IL-12p40 and inducible nitric oxide synthase (iNOS) mRNA expression in freshly isolated TSC1KO peritoneal macrophages as compared with WT macrophages ( P <0.01, Fig. 2a ). Consistently, more TNF-α, IL-12p70 and NO were produced by TSC1KO macrophages than WT macrophages as determined by enzyme-linked immunosorbent assay and biochemical assays ( Fig. 2b,c ). Macrophages derived from bone marrow cells induced by M-CSF in vitro also expressed more TNF-α and IL-12 compared with WT cells after LPS stimulation ( Supplementary Fig. 3 ). TSC1KO macrophages expressed high levels of p-S6 (235/236), the downstream marker of mTOR signalling [17] , [34] , when detected by western blots ( Supplementary Fig. 4 ). However, when freshly isolated peritoneal macrophages were used to investigate the possible role of mTOR in the TSC1/2-mediated regulation of TNF-α and IL-12 production, we found that blocking mTOR with low and high doses of Rapa for 90-min pretreatment failed to inhibit the enhanced TNF-α and IL-12 production in TSC1-deficient macrophages at both mRNA and protein levels ( Fig. 2d,e ), although Rapa completely blocked p-S6 (235/236) levels induced by LPS ( Fig. 2f ). Instead, Rapa treatment at low doses somewhat elevated TNF-α and IL-12 mRNA expression ( P <0.01, Fig. 2d ). Macrophages isolated from WT and TSC1KO mice pretreated with Rapa (50 μg kg −1 body weight) in vivo for 3 days showed enhanced TNF-α, IL-12 and iNOS expression in both mRNA and protein levels after LPS stimulation ( Fig. 2g , Supplementary Fig. 5 ). To further demonstrate the role of mTOR in the enhanced inflammatory response of TSC1KO macrophages, we produced mice with mTOR deletion ( LysMCremTOR loxp/loxp ; herein referred to as mTORKO) or with TSC1 and mTOR double deletion ( LysMCreTSC1 loxp/loxp /mTOR loxp/loxp ; herein referred to as TSC1/mTORKO) in myeloid cells. Macrophages with mTOR deletion expressed higher levels of TNF-α, IL-12p40 and iNOS compared with WT cells after LPS or LPS/IFN-γ stimulation ( P <0.01, Supplementary Fig. 6 ). Peritoneal macrophages isolated from TSC1/mTORKO mice expressed significantly higher levels of TNF-α, IL-12p40 and iNOS compared with WT cells after LPS stimulation as determined by real-time PCR and intracellular staining flow cytometry assays ( P <0.01, Fig. 2h , and Supplementary Fig. 7 ), Importantly, deletion of mTOR failed to reverse and in fact further promoted the enhanced TNF-α, IL-12p40 and iNOS expression of TSC1KO macrophages after LPS stimulation ( P <0.01, Fig. 2h ). These results collectively indicate that TSC1 inhibits inflammatory M1 polarization in an mTOR-independent manner. The increased mTOR activity caused by TSC1 deficiency in macrophages might even inhibit the inflammatory response to LPS and LPS/IFN-γ. 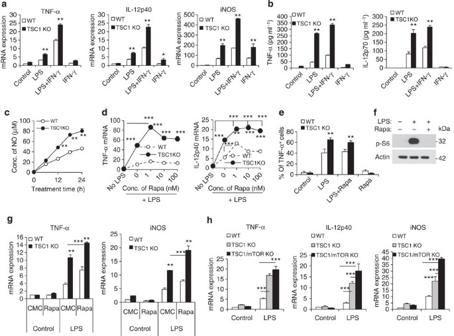Figure 2: TSC1-deficient macrophages are hypersensitive to LPS and LPS plus IFN-γ stimulation. (a) The peritoneal macrophages were stimulated with LPS or LPS+IFN-γ for 6 h and the expression of TNF-α, IL-12 and iNOS was determined by real-time PCR. (b) The freshly isolated peritoneal macrophages were stimulated with LPS or LPS+IFN-γ for 6 h. The levels of TNF-α and IL-12p70 in the culture medium were determined by enzyme-linked immunosorbent assay. (c) Macrophages were stimulated with LPS+IFN-γ for 6 h and the NO levels in the culture medium were detected. (d) Macrophages were pretreated with the indicated doses of Rapa for 90 min and then stimulated with LPS for 6 h. TNF-α and IL-12 mRNA expressions were determined by real-time PCR. (e) Macrophages were pretreated with Rapa (100 nM) for 90 min and then stimulated with LPS for 6 h. TNF-α expression was determined by intracellular staining flow cytometry. (f) The WT peritoneal macrophages were pretreated with Rapa for 90 min and were then treated with LPS for an additional 30 min. The p-S6 activity was detected using western blots. (g) WT and TSC1KO mice were treated with Rapa (50 μg kg−1) for 3 days. The freshly isolated peritoneal macrophages were treated with LPSin vitrofor 6 h, and the TNF-α and iNOS mRNA expressions were determined by real-time PCR. (h) The freshly isolated peritoneal macrophages were treated with LPSin vitrofor 6 h. Assays were performed more than two times. Data were shown as mean±s.d. (N=5). *P<0.05, **P<0.01, ***P<0.001 compared with WT mice or between the indicated groups.Pvalues were determined using Student’st-tests. Images have been cropped for presentation; full-size blot is shown inSupplementary Fig. 24. Figure 2: TSC1-deficient macrophages are hypersensitive to LPS and LPS plus IFN-γ stimulation. ( a ) The peritoneal macrophages were stimulated with LPS or LPS+IFN-γ for 6 h and the expression of TNF-α, IL-12 and iNOS was determined by real-time PCR. ( b ) The freshly isolated peritoneal macrophages were stimulated with LPS or LPS+IFN-γ for 6 h. The levels of TNF-α and IL-12p70 in the culture medium were determined by enzyme-linked immunosorbent assay. ( c ) Macrophages were stimulated with LPS+IFN-γ for 6 h and the NO levels in the culture medium were detected. ( d ) Macrophages were pretreated with the indicated doses of Rapa for 90 min and then stimulated with LPS for 6 h. TNF-α and IL-12 mRNA expressions were determined by real-time PCR. ( e ) Macrophages were pretreated with Rapa (100 nM) for 90 min and then stimulated with LPS for 6 h. TNF-α expression was determined by intracellular staining flow cytometry. ( f ) The WT peritoneal macrophages were pretreated with Rapa for 90 min and were then treated with LPS for an additional 30 min. The p-S6 activity was detected using western blots. ( g ) WT and TSC1KO mice were treated with Rapa (50 μg kg −1 ) for 3 days. The freshly isolated peritoneal macrophages were treated with LPS in vitro for 6 h, and the TNF-α and iNOS mRNA expressions were determined by real-time PCR. ( h ) The freshly isolated peritoneal macrophages were treated with LPS in vitro for 6 h. Assays were performed more than two times. Data were shown as mean±s.d. ( N =5). * P <0.05, ** P <0.01, *** P <0.001 compared with WT mice or between the indicated groups. P values were determined using Student’s t -tests. Images have been cropped for presentation; full-size blot is shown in Supplementary Fig. 24 . Full size image TSC1/2 inhibits M1 polarization via direct action on Ras LPS activates several signalling pathways including NF-κB, ERK, JNK, PI3K/AKT cascade, p38 MAPK, as well as signal transducer and activator of transcription signals in macrophages [35] , [36] , [37] . The intracellular signals of TLR4 were detected using western blot assays. LPS induced p38 MAPK, MEK–ERK, JNK, NF-κB and AKT activation by phosphorylation in both WT and TSC1KO peritoneal macrophages ( Fig. 3a ). However, enhanced MEK1/2 and ERK activities were striking in TSC1KO macrophages compared with WT macrophages after LPS stimulation ( Fig. 3a ), whereas TSC1-deficient macrophages displayed identical levels of p-p38 MAPK, p-STAT1, p-JNK, p-IKKα/β and p-p65 as WT macrophages after LPS stimulation ( Fig. 3a,b ). In contrast, TSC1KO macrophages had poor p-AKT (Thr308, Ser473) activation during LPS response compared with WT macrophages ( Fig. 3a ), likely due to the enhanced mTOR activity caused by TSC1 deficiency ( Supplementary Fig. 4 ) in agreement with the previous studies [13] , [38] . To explore the possible role of ERK in mediating the inhibitory role of TSC1 in macrophage inflammation, we employed the specific MEK1/2 inhibitor PD98059 to block ERK pathway. Blocking ERK significantly rescued the enhanced TNF-α and IL-12 production in TSC1-deficient macrophages after LPS stimulation ( Fig. 3c,d , and Supplementary Fig. 8 ), indicating that ERK activity is involved in TSC1 regulation of macrophage inflammation. Further studies demonstrated that the increased p-ERK activity in TSC1-deficient macrophages was independent of mTOR and PI3K pathways, as inhibition of mTOR and PI3K by their specific chemical inhibitors Rapa and LY294002, respectively, failed to alter p-ERK activation in LPS-stimulated macrophages ( Fig. 3e , and Supplementary Fig. 9 ). The freshly isolated peritoneal macrophages from TSC1KO mice, which were pretreated with Rapa (50 μg kg −1 ) for 3 days, had similar ERK activity as macrophages of Rapa-untreated TSC1KO mice, but still had enhanced ERK activity compared with WT macrophages after LPS stimulation ( Fig. 3f ). Furthermore, macrophages derived from mTORKO bone marrow cells had similar levels of ERK activity as WT cells after LPS stimulation in vitro ( Fig. 3g ). It is known that TSC2 contains a GAP domain that stimulates the intrinsic GTPase activity of Rheb, thereby enhancing the conversion of Rheb into its GDP-bound inactive state [39] . Therefore, the enhanced MEK and ERK activities that are mTOR-independent promoted us to explore whether TSC2 directly acts on Ras GTPase in a negative manner. To determine whether TSC2 directly acts on Ras GTPase, we performed molecular mechanism studies using TSC2KO MEFs ( Supplementary Fig. 10 ). GST pull-down assay showed that GTP-bound Ras GTPase increased in TSC2 KO MEF cells compared with WT cells ( Fig. 3h ), supporting the notion that TSC1/2 may inhibit Ras GTPase. Indeed, the in vitro biochemical assays using purified TSC2 and Ras GTPase proteins clearly showed that TSC2 could directly interact with Ras GTPase and subsequently inhibit Ras GTPase activity ( Fig. 3i ). In parallel with studies of MEFs, GTP-bound Ras GTPase in TSC1KO macrophages were also increased compared with WT macrophages, no matter if cells were stimulated with LPS or not ( Fig. 3j ), indicating the enhanced Ras GTPase activity in TSC1KO macrophages. Thus, we identified Ras GTPase as a direct target molecule of TSC2. The inhibition of TSC1/2 on Ras GTPase activity downregulates the Raf1–MEK–ERK–M1 polarization pathway. In contrast, TSC1/2 complex deficiency in macrophages resulted in high Ras GTPase activity, and consequently, high MEK–ERK activation promoted inflammatory M1 polarization. 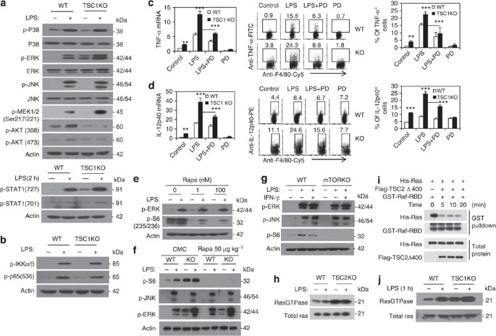Figure 3: The hypersensitivity to LPS of TSC1KO macrophages is mediated by TSC1/2-Ras–ERK. (a) The activity of p38 MAPK, ERK, JNK, MEK, AKT, STAT1 in both WT and TSC1KO peritoneal macrophages after LPS (100 ng ml−1) treatment were detected by western blotting. (b) The levels of p-IKK and p-p65 in WT and TSC1KO macrophages after LPS (100 ng ml−1) treatment were detected by western blotting. Experiments showing identical results were performed two times. (c,d) Inhibition of ERK by PD98059 (50 μM) significantly rescued the enhanced TNF-α and IL-12 expression in TSC1KO macrophages after LPS (100 ng ml−1) treatment for 6 h as determined by real-time PCR and intracellular staining flow cytometry. Data were shown as mean±s.d. (N=5). **P<0.01, ***P<0.001 compared with WT control mice. (e) WT macrophages were pretreated with Rapa (100 nM) for 90 min and then stimulated with LPS for 30 min. The p-ERK and p-S6 levels were determined by western blots. (f) WT and TSC1KO mice were treated with Rapa (50 μg kg−1) for 3 days. The isolated peritoneal macrophages were treated with LPSin vitrofor 30 min and the p-S6, p-JNK, p-ERK and β-actin protein levels were determined by western blots. (g) The p-ERK and p-JNK activity in WT and mTORKO macrophages after LPS or LPS+IFN-γ treatment was determined by western blots. (h) Ras GTPase activity in WT and TSC2KO MEFs was detected as described in materials and methods. (i) TSC2 acted as a GAP towards Ras GTPasein vitroas detected by chemical assays. (j) WT and TSC1KO bone marrow-derived macrophages by M-CSF were stimulated with LPS for 1 h and the GTP-bound Ras amount was determined as described in the methods. Experiments were done more than two times.Pvalues were determined using Student’st-tests. Images have been cropped for presentation; full-size blot is shown inSupplementary Fig. 25. Figure 3: The hypersensitivity to LPS of TSC1KO macrophages is mediated by TSC1/2-Ras–ERK. ( a ) The activity of p38 MAPK, ERK, JNK, MEK, AKT, STAT1 in both WT and TSC1KO peritoneal macrophages after LPS (100 ng ml −1 ) treatment were detected by western blotting. ( b ) The levels of p-IKK and p-p65 in WT and TSC1KO macrophages after LPS (100 ng ml −1 ) treatment were detected by western blotting. Experiments showing identical results were performed two times. ( c , d ) Inhibition of ERK by PD98059 (50 μM) significantly rescued the enhanced TNF-α and IL-12 expression in TSC1KO macrophages after LPS (100 ng ml −1 ) treatment for 6 h as determined by real-time PCR and intracellular staining flow cytometry. Data were shown as mean±s.d. ( N =5). ** P <0.01, *** P <0.001 compared with WT control mice. ( e ) WT macrophages were pretreated with Rapa (100 nM) for 90 min and then stimulated with LPS for 30 min. The p-ERK and p-S6 levels were determined by western blots. ( f ) WT and TSC1KO mice were treated with Rapa (50 μg kg −1 ) for 3 days. The isolated peritoneal macrophages were treated with LPS in vitro for 30 min and the p-S6, p-JNK, p-ERK and β-actin protein levels were determined by western blots. ( g ) The p-ERK and p-JNK activity in WT and mTORKO macrophages after LPS or LPS+IFN-γ treatment was determined by western blots. ( h ) Ras GTPase activity in WT and TSC2KO MEFs was detected as described in materials and methods. ( i ) TSC2 acted as a GAP towards Ras GTPase in vitro as detected by chemical assays. ( j ) WT and TSC1KO bone marrow-derived macrophages by M-CSF were stimulated with LPS for 1 h and the GTP-bound Ras amount was determined as described in the methods. Experiments were done more than two times. P values were determined using Student’s t -tests. Images have been cropped for presentation; full-size blot is shown in Supplementary Fig. 25 . Full size image TSC1 controls M2 polarization via mTOR-dependent C/EBPβ The role of TSC1/2 complex in IL-4-induced M2 polarization has been recently demonstrated [32] . After IL-4 stimulation, TSC1-deficient peritoneal macrophages expressed reduced arginase 1 (Arg1), found in inflammatory zone 1 (Fizz1), and chitinase 3-like-3/Ym1), hallmarks of M2 macrophages [40] , as determined by quantitative PCR and western blots ( P <0.001, Fig. 4a and Supplementary Fig. 11A ). The decreased M2 polarization was also observed in the in vitro -derived macrophages of TSC1KO bone marrow cells ( Supplementary Fig. 11B ). 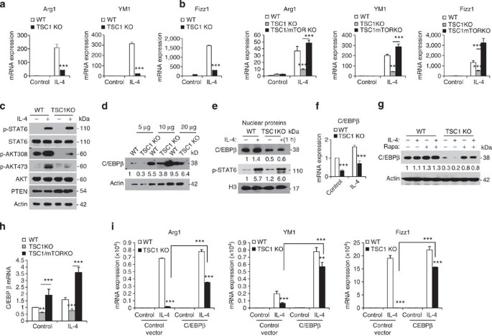Figure 4: The defective response to IL-4 of TSC1KO macrophages is mediated by mTOR-C/EBPβ. (a) The Arg1, Fizz1 and Ym1 mRNA expressions in WT and TSC1KO peritoneal macrophages were determined by real-time PCR after IL-4 stimulation for 48 h. (b) The Arg1, Fizz1 and Ym1 mRNA expressions in WT, TSC1KO and TSC1/mTORKO peritoneal macrophages were determined by real-time PCR after IL-4 stimulation for 48 h. (c) The levels of p-STAT6, STAT6, p-AKT308, p-AKT473, AKT, pTEN and β-actin in WT and TSC1KO macrophages after IL-4 (1,000 U ml−1) treatment were detected by western blots. (d) C/EBPβ expression in WT and TSC1KO peritoneal macrophages was determined by western blots. (e) The levels of C/EBPβ, p-STAT6 and loading control protein H3 in the nuclear proteins of WT and TSC1KO macrophages after IL-4 (1,000 U ml−1) treatment were detected by western blots. (f) C/EBPβ expression in WT and TSC1KO peritoneal macrophages was determined by real-time PCR. (g) WT and TSC1KO peritoneal macrophages were pretreated with Rapa (100 nM) for 1 h and then stimulated with IL-4 for an additional 72 h. The C/EBPβ expression was determined by western blots. (h) Deletion of mTOR reverses the decreased C/EBPβ expression in TSC1KO peritoneal macrophages as determined by real-time PCR. (i) G-CSF-induced bone marrow-derived macrophages were used to overexpress C/EBPβ and the IL-4-induced M2 polarization was done as described in methods. Data (ina,b,f,h,i) were shown as mean±s.d. (N=5). **P<0.01, ***P<0.001 compared with WT control mice or the indicated groups.Pvalues were determined using Student’st-tests. Experiments showing identical results were performed at least twice. Images have been cropped for presentation; full-size blot is shown inSupplementary Fig. 26. Figure 4: The defective response to IL-4 of TSC1KO macrophages is mediated by mTOR-C/EBPβ. ( a ) The Arg1, Fizz1 and Ym1 mRNA expressions in WT and TSC1KO peritoneal macrophages were determined by real-time PCR after IL-4 stimulation for 48 h. ( b ) The Arg1, Fizz1 and Ym1 mRNA expressions in WT, TSC1KO and TSC1/mTORKO peritoneal macrophages were determined by real-time PCR after IL-4 stimulation for 48 h. ( c ) The levels of p-STAT6, STAT6, p-AKT308, p-AKT473, AKT, pTEN and β-actin in WT and TSC1KO macrophages after IL-4 (1,000 U ml −1 ) treatment were detected by western blots. ( d ) C/EBPβ expression in WT and TSC1KO peritoneal macrophages was determined by western blots. ( e ) The levels of C/EBPβ, p-STAT6 and loading control protein H3 in the nuclear proteins of WT and TSC1KO macrophages after IL-4 (1,000 U ml −1 ) treatment were detected by western blots. ( f ) C/EBPβ expression in WT and TSC1KO peritoneal macrophages was determined by real-time PCR. ( g ) WT and TSC1KO peritoneal macrophages were pretreated with Rapa (100 nM) for 1 h and then stimulated with IL-4 for an additional 72 h. The C/EBPβ expression was determined by western blots. ( h ) Deletion of mTOR reverses the decreased C/EBPβ expression in TSC1KO peritoneal macrophages as determined by real-time PCR. ( i ) G-CSF-induced bone marrow-derived macrophages were used to overexpress C/EBPβ and the IL-4-induced M2 polarization was done as described in methods. Data (in a , b , f , h , i ) were shown as mean±s.d. ( N =5). ** P <0.01, *** P <0.001 compared with WT control mice or the indicated groups. P values were determined using Student’s t -tests. Experiments showing identical results were performed at least twice. Images have been cropped for presentation; full-size blot is shown in Supplementary Fig. 26 . Full size image IL-4R expression on peritoneal macrophages was assessed using flow cytometry. Surprisingly, the CD124 expression was enhanced in TSC1KO macrophages compared with WT macrophages ( Supplementary Fig. 12 ), excluding the possibility that the poor IL-4-induced M2 polarization of TSC1KO macrophages is due to IL-4R expression defects. To clarify the intracellular pathways involved in TSC1/2-mediated M2 polarization, we studied whether or not mTOR is required. Blocking mTOR activity by its specific inhibitor Rapa almost completely rescued the M2 differentiation deficiency of TSC1KO macrophages as indicated by the enhanced Arg1, Fizz1 and Ym1 expression in Rapa-treated TSC1KO macrophages, regardless of the dosage used ( Supplementary Fig. 13A–C ). On the other hand, macrophages derived from mTORKO bone marrow cells by M-CSF expressed significantly higher levels of Arg1, Ym1 and Fizz1 compared with WT macrophages after IL-4 stimulation ( Supplementary Fig. 13D ). Furthermore, deletion of mTOR significantly reversed the decreased Arg1, Ym1 and Fizz1 expression in IL-4-stimulated TSC1KO macrophages as determined by real-time PCR ( Fig. 4b ). Therefore, these studies confirm that the enhanced mTOR activity is certainly involved in the poor M2 polarization of TSC1KO macrophages. It is well known that STAT6 and C/EBPβ play a central role in IL-4-induced M2 macrophage polarization [9] , [41] . After IL-4 treatment, TSC1KO peritoneal macrophages had identical levels of p-STAT6 activity relative to WT macrophages, but TSC1KO macrophages had markedly reduced p-AKT (Thr 308 , Ser 473 ) activity and nuclear C/EBPβ protein expression than WT macrophages ( Fig. 4c–e ). The decreased C/EBPβ expression in TSC1KO macrophages was further confirmed by real-time PCR ( P <0.01, Fig. 4f ). Interestingly, Rapa treatment for 72 h markedly reversed the impaired C/EBPβ expression in TSC1KO macrophages ( Fig. 4g ). Macrophages derived from mTORKO bone marrow cells expressed more C/EBPβ than WT macrophages as determined by western blots ( Supplementary Fig. 14 ). Importantly, deletion of mTOR significantly reversed the decreased C/EBPβ expression in TSC1KO peritoneal macrophages as determined by real-time PCR ( P <0.01, Fig. 4h ). To see whether the decreased C/EBPβ expression is involved in the poor M2 polarization of TSC1KO macrophages, we overexpressed C/EBPβ in WT and TSC1KO bone marrow cell-derived macrophages ( Supplementary Fig. 15 ). Overexpression of C/EBPβ significantly rescued the decreased Arg1, Ym1 and Fizz1 expression in TSC1KO macrophages ( P <0.01, Fig. 4i ). These results collectively suggest that the decreased C/EBPβ expression in TSC1KO macrophages is induced by the overactivated mTOR activity and is involved in the poor M2 polarization. In addition, considering that TSC1KO macrophages had high ERK activity, we investigated whether ERK participates in regulating C/EBPβ expression and M2 polarization. Inhibiting ERK had no effect on C/EBPβ expression in TSC1KO macrophages even when the cells were pretreated with PD98059, the inhibitor of ERK, for 72 h ( Supplementary Fig. 16A ). Meanwhile, PD98059 did not show a significant impact on the Arg1, Ym1 and Fizz1 expression in TSC1KO macrophages ( P >0.05, Supplementary Fig. 16B ). Therefore, the enhanced ERK activity is not involved in the poor M2 polarization of TSC1KO macrophages. TSC1KO mice spontaneously develop inflammatory disorder Four-to-five week-old TSC1-deficient mice had normal thymocyte development and undetectable changes in the percentages and cell numbers of CD4 + T cells, CD8 + T cells, B cells, monocytes, DCs, natural killer) cells and granulocytes in peripheral blood, spleen, peripheral lymph nodes), mesenteric LNs (mLNs) and bone marrow ( Supplementary Fig. 17 ). These data indicate that TSC1 deficiency, specifically in myeloid cells, does not impair the development of innate cells including monocytes, DCs, NKs and granulocytes at an early age. The TSC1KO mice displayed no gross abnormalities within 6 weeks of birth. Astonishingly, more and more TSC1KO mice died as early as 10 weeks after birth, whereas all the WT littermates survived well without clinical abnormalities ( P <0.001, Fig. 5a ). These mice generally started losing body weight ( P <0.01, Fig. 5b ). Macroscopic examination found that intestines from sick TSC1KO mice showed massive haemorrhaging ( Supplementary Fig. 18 ). Histological analysis revealed a typical but severe destructive inflammatory response in the colon, liver and lungs of TSC1KO mice, including massive inflammatory infiltrates ( Supplementary Fig. 19 ). Meanwhile, the spleen, pLNs and mLNs were larger in sick TSC1KO mice than WT littermates ( Fig. 5c ). High levels of TNF-α and IL-12p40 were detected in the sera of ill TSC1KO mice relative to the age-matched WT mice ( P <0.01, Fig. 5d ). Moreover, the activating CD4 + CD25 + Foxp3 − T effector cells were significantly higher in the spleens of TSC1KO mice when compared with WT littermates ( P <0.01, Fig. 5e ). Consistently, more memory/activated CD4 + CD62L − CD44 high T cells and less naïve CD4 + CD62L + CD44 low T cells in the spleens and mLNs were observed in sick TSC1KO mice than WT mice ( P <0.05 or P <0.001, Fig. 5f ). Freshly isolated macrophages from sick TSC1KO mice displayed higher levels of CD80, CD86 and CD54 expression, indicating the potential activation status of macrophages in vivo ( Fig. 5g ). Furthermore, expression of TNF-α and IL-12 in the lungs, liver and colons of sick TSC1KO mice was significantly higher than WT mice as determined by quantitative PCR ( P <0.05 or P <0.001, Fig. 5h ). These data collectively indicate that myeloid cell-specific TSC1KO mice are highly susceptible to an autoinflammatory syndrome. 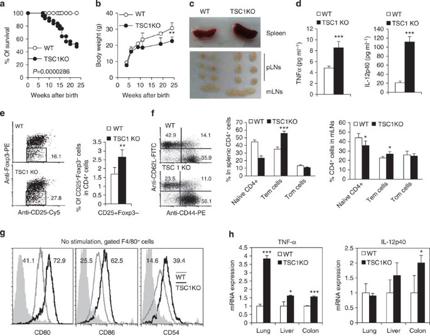Figure 5: Mice with a myeloid-specific TSC1 deficiency suffer from inflammatory disorders. (a) Kaplan–Meier plots of WT and TSC1KO mouse survival after birth were shown.Pvalues were determined using Log-rank tests. (b) The body weight of both WT and TSC1KO mice after birth were summarized. (c) Spleens and LNs of TSC1KO and WT littermates. (d) TNF-α and IL-12 levels in the sera of sick TSC1KO mice were measured by enzyme-linked immunosorbent assay. (e) Fluorescence-activated cell sorting (FACS) analysis of CD4+CD25+Foxp3−T cells in TSC1KO mice suffering from an autoinflammatory disorder compared with WT mice. (f) FACS analysis of memory/activated CD4+CD62LlowCD44highT cells and naïve CD4+T cells in the spleens and LNs of TSC1KO and WT mice. (g) Primary macrophages freshly isolated from the peritoneal cavity of TSC1KO mice were assayed for CD80, CD86 and CD54 levels by flow cytometry. The median fluorescence intensity of each sample was shown in the panels. (h) The TNF-α and IL-12 expressions in lung, liver and colon tissues were detected using real-time PCR assays. Eighteen mice in each group were observed for survival and body weight (a,b). In other assays, more than five mice in each group were assayed. Data were shown as mean±s.d. *P<0.05, **P<0.01, ***P<0.001 compared with WT control mice.Pvalues were determined using Student’st-tests. Figure 5: Mice with a myeloid-specific TSC1 deficiency suffer from inflammatory disorders. ( a ) Kaplan–Meier plots of WT and TSC1KO mouse survival after birth were shown. P values were determined using Log-rank tests. ( b ) The body weight of both WT and TSC1KO mice after birth were summarized. ( c ) Spleens and LNs of TSC1KO and WT littermates. ( d ) TNF-α and IL-12 levels in the sera of sick TSC1KO mice were measured by enzyme-linked immunosorbent assay. ( e ) Fluorescence-activated cell sorting (FACS) analysis of CD4 + CD25 + Foxp3 − T cells in TSC1KO mice suffering from an autoinflammatory disorder compared with WT mice. ( f ) FACS analysis of memory/activated CD4 + CD62L low CD44 high T cells and naïve CD4 + T cells in the spleens and LNs of TSC1KO and WT mice. ( g ) Primary macrophages freshly isolated from the peritoneal cavity of TSC1KO mice were assayed for CD80, CD86 and CD54 levels by flow cytometry. The median fluorescence intensity of each sample was shown in the panels. ( h ) The TNF-α and IL-12 expressions in lung, liver and colon tissues were detected using real-time PCR assays. Eighteen mice in each group were observed for survival and body weight ( a , b ). In other assays, more than five mice in each group were assayed. Data were shown as mean±s.d. * P <0.05, ** P <0.01, *** P <0.001 compared with WT control mice. P values were determined using Student’s t -tests. Full size image Sensitivity of TSC1KO mice to M1 and M2-releated diseases To further determine the impact of macrophages in vivo in TSC1KO mice, we used an acute endotoxin shock model [42] . After WT and TSC1KO mice received a low dose of LPS (5 mg kg −1 body weight), WT mice survived well for at least 3 days, but all TSC1KO mice died within 24 h ( P <0.001, Fig. 6a ). Pathological tests found that the liver and kidneys of LPS-treated TSC1KO mice had immune cell infiltration and massive haemorrhaging ( Fig. 6b and Supplementary Fig. 20A ). Clinical tests revealed significantly higher levels of alanine aminotransferase and aspartate aminotransferase in the sera of LPS-treated TSC1KO mice compared with LPS-treated WT mice ( P <0.01, Fig. 5c ). Accordingly, the plasma levels of inflammatory cytokines TNF-α and IL-12 were significantly higher in TSC1KO mice than WT mice after LPS challenge as detected by enzyme-linked immunosorbent assay assays ( P <0.001, Fig. 5d , Supplementary Fig. 20B ). Furthermore, a lower dose of LPS (2.5 mg kg −1 body weight) also induced more severe inflammatory response and tissue damage in TSC1KO mice compared with WT mice ( Supplementary Fig. 21 ). These results indicate that TSC1 deficiency predisposes mice to M1-mediated pathology in vivo . 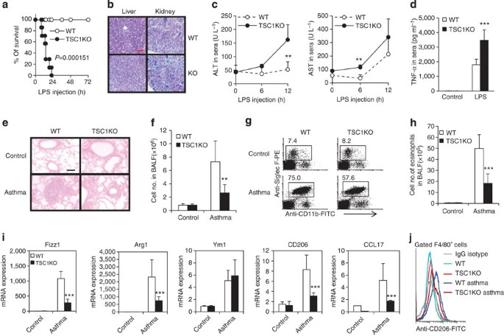Figure 6: Mice with a myeloid-specific TSC1 deficiency are sensitive to LPS and resistant to OVA-induced asthma. (a) Kaplan–Meier plots of WT and TSC1KO mouse survival after LPS injection (5 mg kg−1body weight) were shown.Pvalues were determined using Log-rank tests. (b) Hematoxylin and eosin stain (H&E) staining of liver and kidney tissues from LPS-treated WT and TSC1KO mice was presented. Scale bar, 100 μM. (c) The levels of alanine aminotransferase (ALT) and aspartate aminotransferase (AST) in the sera of WT and TSC1KO mice after LPS treatment were shown. (d) TNF-α concentration was measured in the sera of TSC1KO and WT mice 2 h after LPS injection. (e) H&E staining of lung tissues of OVA-challenged or control WT and TSC1KO miceAQ were presented. OVA-presensitized WT and TSC1KO mice were challenged with aerosolized OVA daily for 5 days as described in materials and methods. The assays were performed on day 6 after OVA challenge. Scale bar, 100 μM. (f) BALF cell numbers in TSC1KO and WT mice after OVA challenge. (g) The infiltrated CD11b+Siglec F+granulocytes in BALF of control and OVA-challenged mice were assayed by flow cytometry. (h) Eosinophil numbers in BALF of TSC1KO mice and WT mice after OVA challenge. (i) The mRNA expressions of Fizz1, Arg1, Ym1, CD206 and CCL17 in macrophages isolated from BALF of WT and TSC1KO mice regardless of OVA challenge were detected by real-time PCR. (j) Macrophages isolated from BALF of OVA-challenged TSC1KO and WT mice were analysed by multicolor flow cytometry. Each assay was performed more than two times. Data were shown as mean±s.d. (N=6). *P<0.05, **P<0.01, ***P<0.001 compared with WT control mice.Pvalues were determined using Student’st-tests. Figure 6: Mice with a myeloid-specific TSC1 deficiency are sensitive to LPS and resistant to OVA-induced asthma. ( a ) Kaplan–Meier plots of WT and TSC1KO mouse survival after LPS injection (5 mg kg −1 body weight) were shown. P values were determined using Log-rank tests. ( b ) Hematoxylin and eosin stain (H&E) staining of liver and kidney tissues from LPS-treated WT and TSC1KO mice was presented. Scale bar, 100 μM. ( c ) The levels of alanine aminotransferase (ALT) and aspartate aminotransferase (AST) in the sera of WT and TSC1KO mice after LPS treatment were shown. ( d ) TNF-α concentration was measured in the sera of TSC1KO and WT mice 2 h after LPS injection. ( e ) H&E staining of lung tissues of OVA-challenged or control WT and TSC1KO miceAQ were presented. OVA-presensitized WT and TSC1KO mice were challenged with aerosolized OVA daily for 5 days as described in materials and methods. The assays were performed on day 6 after OVA challenge. Scale bar, 100 μM. ( f ) BALF cell numbers in TSC1KO and WT mice after OVA challenge. ( g ) The infiltrated CD11b + Siglec F + granulocytes in BALF of control and OVA-challenged mice were assayed by flow cytometry. ( h ) Eosinophil numbers in BALF of TSC1KO mice and WT mice after OVA challenge. ( i ) The mRNA expressions of Fizz1, Arg1, Ym1, CD206 and CCL17 in macrophages isolated from BALF of WT and TSC1KO mice regardless of OVA challenge were detected by real-time PCR. ( j ) Macrophages isolated from BALF of OVA-challenged TSC1KO and WT mice were analysed by multicolor flow cytometry. Each assay was performed more than two times. Data were shown as mean±s.d. ( N =6). * P <0.05, ** P <0.01, *** P <0.001 compared with WT control mice. P values were determined using Student’s t -tests. Full size image In an ovalbumin (OVA)-induced allergic asthma mouse model, in which M2 macrophages play a critical role as shown before [7] , [43] , [44] , we found that TSC1KO mice were resistant to OVA-induced asthma as determined by reduced pathological changes, significantly less infiltration by leukocytes and eosinophils in the bronchoalveolar lavage fluid (BALF) of TSC1KO mice than that in WT mice after OVA challenge ( Fig. 6e–h ). Moreover, the freshly isolated macrophages from the BALF of TSC1KO asthma mice expressed significantly less Fizz1, Arg1, CCL17 and CD206, markers of M2-polarized macrophages [35] , as detected by quantitative PCR ( P <0.001, Fig. 6i ). Freshly isolated alveolar macrophages from OVA-challenged WT mice expressed more CD206 molecules than macrophages isolated from OVA-unchallenged WT mice, but macrophages from OVA-challenged TSC1KO mice displayed lower levels of CD206 expression compared with those from OVA-challenged WT mice ( Fig. 6j ). Thus, deficiency of TSC1 prevents M2 polarization in vivo and reduces M2-mediated disease. Macrophages influence the quality, duration and magnitude of innate immune responses as well as balance the anti-pathogen response and potential tissue injury [35] . It is well known that macrophages can be polarized into inflammatory M1 and anti-inflammatory M2 phenotypes, depending on the cytokine milieu. M1 and M2 macrophages differentially express a variety of effector molecules including iNOS, Arg1, Ym1 and Fizz1 (refs 3 , 9 , 45 ) that have distinct impact on inflammatory outcomes. In the present study, we demonstrated that TSC1/2 complex was a critical regulator that controls macrophage polarization via different signalling pathways ( Supplementary Fig. 22 ). Mice with a myeloid cell-specific TSC1 deficiency spontaneously suffered from an autoimmune syndrome, were hypersensitive to endotoxin stress, and were resistant to OVA-induced allergic asthma. Thus, TSC1 is critical for M2 polarization and is capable of attenuating M1 reactions. This unique behaviour pattern led us to conclude that TSC1 is essential for maintaining macrophage homeostasis to prevent spontaneous inflammatory damage in physiological conditions and that TSC1 is one of the key predetermining factors of macrophage polarizing differentiation in pathological cases. TSC1KO mice were hypersensitive to LPS shock; TSC1KO macrophages produced larger amounts of M1-type inflammatory mediators TNF-α, IL-12 and NO for a prolonged period after LPS or LPS plus IFN-γ activation in vitro , indicating that macrophages deficient of TSC1 are highly susceptible to M1 polarization, suggesting that TSC1 is an intrinsic repressor of M1 inflammatory response. The enhanced macrophage inflammatory response in TSC1-deficient mice is consistent with a recent report showing that increased M1 response in TSC1 f/f -ERCre mice, in which TSC1 was deleted via tamoxifen administration for 8 days [31] . However, studies using MEFs and human monocytes showed that deletion of TSC2 decreased the inflammatory response in an mTOR-dependent manner [28] . Our observations in TSC1KO and TSC1/mTORKO macrophages suggest that the enhanced inflammatory response of TSC1-deficient macrophages was not mediated by mTOR pathway, although mTOR inhibition or deletion in macrophages slightly increased inflammatory cytokine production. Actually, the current reports on the roles of TSC1/2-mTOR in the innate inflammation are contradictory. Rapa had different effects on the functions of DCs [22] , [23] , [24] , [25] , [26] . Rapa enhanced inflammatory cytokine production in macrophages via enhancing NF-κB and blocking STAT3 activity [27] , [28] . Rapa significantly blocked the anti-inflammatory effects of glucocorticoids in myeloid immune cells including monocytes and DCs [29] . Rapa treatment enriched NF-kB-related proinflammatory expression pathways and monocyte lineage-specific transcripts in kidney-transplanted recipients [30] . TSC2 −/− mouse embryonic fibroblasts and TSC2-knockdown THP1 cells both expressed less IL-12 and TNF-α but more IL-10 (ref. 28 ). The reasons for this inconsistency are unclear, possibly due to the different cell types and duration of TSC1/2-mTOR inhibition/deletion used in these studies. This will require further clarification in the future. We observed that inhibiting mTOR by Rapa treatment in vitro and in vivo before LPS stimulation or by genetic deletion of mTOR failed to rescue the elevated inflammatory reaction of TSC1KO macrophages. Furthermore, myeloid cell-specific mTOR deletion even led to enhanced M1 function, indicating that mTOR activation inhibits macrophage inflammatory response. Thus, the enhanced M1 differentiation caused by TSC1 deficiency is unlikely to be mediated by mTOR pathways, although mTOR activity was enhanced in TSC1KO macrophages. It is known that the PI3K–AKT kinase signalling pathway plays an important feedback role in LPS-induced macrophage activation [46] . LPS activated PI3K, AKT, ERK, JNK and NF-kB pathways in both WT and TSC1KO macrophages. After LPS stimulation, however, TSC1KO macrophages showed decreased AKT activity, enhanced MEK–ERK activity and similar JNK and NF-kB activity relative to WT macrophages. We did not detect a difference for JNK activation in WT and TSC1KO macrophages after LPS stimulation. Blocking JNK activity did not significantly rescue the elevated TNF-α and IL-12 expressions in LPS-stimulated TSC1KO macrophages. Instead, using a series of biochemical studies, we demonstrated that Ras GTPase is a direct target molecule of TSC2. TSC2 can directly interact with Ras GTPase to promote the conversion of GTP-bound active Ras GTPase into its GDP-bound inactive state. Thus, TSC2 directly inhibits Ras GTPase activity, and in turn, downregulates the Raf-MEK–ERK-TNF-α/IL-12 pathway in macrophages, subsequently inhibiting M1 polarization. Together with the observation that LPS activates AKT and the latter could phosphorylate and inhibit TSC1 (ref. 16 ), our present data provide a new positive feedback regulatory loop, which is constituted of AKT, TSC1/2 complex and Ras GTPase to promote inflammatory response during LPS-induced M1 polarization. Ras–ERK and PI3K–mTOR were originally modelled as linear signalling pathways, but recent data indicate that these pathways often intersect and regulate one another [47] . Direct interaction among TSC2 and Ras GTPase adds one more negative connecting node for the cross-talk between the PI3K–AKT–TSC1/2-mTOR and Ras GTPase–ERK pathways. On the other hand, given that the TSC1/2 complex as well as the Ras GTPase–Raf–MEK–ERK and PI3K–AKT–mTOR pathways are frequently deregulated or mutated in human cancers [48] , we may speculate that the newly identified interaction of TSC2 and Ras GTPase may offer an alternative explanation for the altered Ras GTPase activity in TSC1/2-disregulated tumour cells. Validation in other cells needs to be determined. Th2 cells and IL-4-driven M2 polarization both play active roles in the pathogenesis of allergic asthma [49] . TSC1KO mice were resistant to OVA challenge-induced allergic asthma. As compared with WT controls, TSC1KO mice showed fewer infiltrated immune cells and decreased M2 response. Primary TSC1KO macrophages showed defective M2 polarization as evidenced by poor expression of M2 markers like Arg1, Ym1 and Fizz1 after IL-4 treatment. Thus, TSC1/2 complex is required for M2 macrophage differentiation. Molecular mechanism studies showed that inhibiting mTOR by Rapa almost completely rescued the M2 defects of TSC1KO macrophages, indicating that mTOR is a potent inhibitor of M2 differentiation and blocking mTOR pathway facilitates M2 differentiation. Indeed, mTOR deletion significantly increased M2 hallmarks including Arg1, Fizz1 and Ym1. Deletion of the mTOR gene remarkably reversed otherwise poor M2 polarization in TSC1KO macrophages. In line with the role of TSC1/2 complex on mTOR in other cells [20] , [39] , TSC1KO macrophages also displayed enhanced mTOR activity. Further studies showed that activated mTOR in macrophages significantly inhibited the expression of C/EBPβ, which is essential for IL-4-induced M2 polarization [50] . Overexpression of C/EBPβ significantly reversed the poor M2 polarization of TSC1KO macrophages. These data indicate that the M2 differentiation deficiency of TSC1KO macrophages is, at least partially, mediated by the mTOR-C/EBPβ pathway. Both appropriate feedback inhibitory loops to limit macrophage inflammatory activity and the balance of M1/M2 polarization are critical for maintaining host macrophage homeostasis [51] . Myeloid cell-specific TSC1KO mice spontaneously develop an inflammatory disorder, as evidenced by the pathological alterations of liver, intestine and lung, impaired liver function, increased inflammatory cytokines, as well as elevated T-cell and macrophage activation. These results indicate that the TSC1/2 complex is an essential repressor for macrophage activation, M1 polarization and tissue inflammation under physiological conditions. Autoimmune diseases are generally thought to be triggered by aggressive responses of the adaptive immune system to self-antigens. However, accumulating data show that autoimmune diseases like systemic lupus erythematosus can be triggered and accelerated by innate immune cells including macrophages even in the absence of adaptive immune cells like B and T cells [5] , [6] . The present observation showing the autoimmune-like syndrome in mice with a myeloid cell-specific TSC1 deficiency also highlights the critical roles of innate cells in the initiation and progression of autoimmune diseases. In summary, we demonstrate that the TSC1/2 complex directly suppresses the Ras GTPase pathway to inhibit M1 response, and its essential role in M2 activation is mainly mediated by inhibiting the mTOR pathway. Thus, TSC1/2 complex regulates a key checkpoint in macrophage polarization and homeostasis, and failure to control such pathways in macrophages results in spontaneous inflammatory disorders. The identification of the master role of TSC1-related pathways in macrophage activation provides potential targets for macrophage-directed diagnostic and therapeutic strategies. Animals Myeloid cell-specific TSC1 and mTOR conditional knockout mice ( LysMCreTSC1 loxp/loxp and LysMCremTOR loxp/loxp ) were obtained by crossing TSC1 loxp/loxp and mTOR loxp/loxp mice with mice expressing Cre recombinase under the control of the Lysozyme promoter (LysMCre). LysMCre-negative, TSC1 loxp/loxp and mTOR loxp/loxp littermates served as the control. Four-to-five-week-old mice (male and female) were usually used for the in vitro experiments. TSC1 loxp/loxp mice and TSC2KO MEF cells were the generous gifts of Dr Hongbin Zhang (Institute of Basic Medical Sciences and School of Basic Medicine, Peking Union Medical College and Chinese Academy of Medical Sciences, Beijing, China) [52] , [53] . mTOR loxp/loxp mice were kindly provided by Dr Zhongzhou Yang from Center of Model Animal Research at Nanjing University, China [54] . LysMCre mice were kindly offered by Dr Lianfeng Zhang, Key Laboratory of Human Diseases Comparative Medicine, Ministry of Health; Institute of Laboratory Animal Science, CAMS & PUMC [55] . Primers used to identify genetically modified mice are listed in Table 1 . Six-to-eight-week-old female CD45.1 mice were purchased from Beijing University Experimental Animal Center (Beijing, China). All mice were maintained in a specific pathogen-free facility. All experimental manipulations were undertaken in accordance with the Institutional Guidelines for the Care and Use of Laboratory Animals, Institute of Zoology (Beijing, China). Table 1 Primers used for mice identification. Full size table Reagents Anti-mF4/80-PE-Cy5, anti-mCD11b-PE-Cy5, anti-mCD80-PE, anti-mCD86-FITC, anti-mCD54-FITC, anti-mTNF-α-FITC, anti-mCD14-FITC, anti-mGr1-PE, anti-mCD44-PE, anti-mCD124-PE, anti-mCD206-PE and anti-mSiglec F-PE were purchased from BD Biosciences Pharmingen (San Diego, CA). Anti-mF4/80-FITC was procured from Tianjin Sungene Biotech (Tianjin, China). Anti-mIL-12p40-PE, anti-mCD45.1-PE and anti-mCD45.2-Cy5 were purchased from Biolegend (San Diego, CA). Anti-mCD11c-PE-Cy5, anti-mLy6G-PE, anti-mCD25-PE-Cy5, anti-mFoxp3-PE, anti-mCD4-FITC and anti-mCD62L-FITC were purchased from eBioscience (San Diego, CA). Rapamycin (Rapa; LC Laboratory) was reconstituted in ethanol at 60 mg ml −1 and then diluted with DMSO (Sigma-Aldrich, St Louis, MO) to 60 μg ml −1 . The final concentration of Rapa in the culture system was 100 nM. Bacterial lipopolysaccharide (LPS; E. coli 055:B5) were purchased from Sigma-Aldrich. Recombinant mouse IL-4, IL-10, IL-33, TGF-β and IFN-γ were purchased from PeproTech (Rocky Hill, NJ). Inhibitors of MEK (PD98059, used at 50 μM) were purchased from Sigma-Aldrich. The OVA and Alum were purchased from Sigma-Aldrich and then diluted with phosphate-buffered saline (PBS). The primary antibodies against TSC1, TSC2, p-S6 (Thr421/Ser424), p-S6 (Ser235/236), ERK, p-ERK1/2 (Thr202/Tyr204), JNK, p-JNK (Thr183/Tyr185), P38, p-P38 (Thr180/Tyr182), p-MEK1/2 (Ser217/221), Akt (pan), Akt1, Akt2, p-Akt (Thr308), p-Akt (Ser473), PTEN, STAT6, p-STAT6 (Tyr641), p-STAT1 (Tyr701), p-STAT1 (Ser727) and C/EBPβ, arginase 1 and H3 were purchased from Cell Signaling Technology. All of these antibodies were diluted at 1:1,000 in 5% bovine serum albumin, except for the followings: p-S6 (Thr421/Ser424; 1:4,000), p-Akt (Thr308; 1:500), p-Akt (Ser473; 1:500), H3 (1:3,000). Anti-Ras mAb (1:1,000) was from Epitomics. Anti-β-Actin mAb (1:50,000) was purchased from Sigma-Aldrich. Cell preparation Bone marrow cells were cultured with Dulbecco’s modified Eagle medium (DMEM) containing 10% (v/v) FBS and 10 ng ml −1 of mouse M-CSF or 10 ng ml −1 of mouse GM-CSF for 12 days to obtain bone marrow-derived macrophagess [56] . Primary mouse peritoneal macrophages were obtained from the peritoneal exudates of 4-to-6-week-old mice [57] . The peritoneal exudate cells were washed twice with PBS solution and adjusted to 1 × 10 6 cells ml −1 in DMEM cultured for 3-4 h at 37 °C and 5% CO 2 . The non-adherent cells were removed by washing with warm PBS. The purity of macrophages was analysed by FCM (Beckman, CA), using a mouse macrophage marker F4/80. The adherent cells constituted more than 90% of F4/80 + macrophages. Intracellular cytokine staining Macrophages were stimulated for 6 h with LPS (100 ng ml −1 ) or LPS plus IFN-γ (10 ng ml −1 ) in the presence of GolgiPlug (BD Pharmingen). Cells were fixed and analysed for the intracellular production of cytokines (BD Pharmingen) by staining with anti-mTNF-α-FITC (BD Biosciences Pharmingen, 1:200) and anti-mIL-12p40-PE (Biolegend, 1:200) Abs, respectively and subsequent flow cytometry assay [58] . For the recovery assay, cells were pretreated with PD and Rapa for 30 and 90 min respectively, and then treated with LPS and GolgiPlug for another 6 h. Rapa treatment in vivo Age-matched WT and TSC1KO mice were injected intraperitoneally with Rapa (50 μg kg −1 body weight) or CMC (carboxymethyl cellulose sodium) every day for 3 days. OVA-induced allergic asthma The WT and TSC1 knockout mice were sensitized by two intraperitoneal injections of 10 μg OVA and 1 mg alum at days 1 and 14, whereas control mice were sham sensitized only with PBS [7] . From day 21, mice were challenged 30 min per day with aerosolized OVA (1% w/v) for 5 consecutive days. Mice were assessed 24 h after the last OVA challenge. Blood was obtained from the retroorbital plexus. Cells from BALF were analysed by fluorescence-activated cell sorting with anti-mF4/80, anti-mCD206, anti-mLy6G and anti-mSiglec F mAbs as well as by real-time PCR for detection of M2 markers, including Arg1, Fizz1, Ym1, CCL17 and CD206. Lungs were fixed with formaldehyde and embedded in paraffin. Thin sections of the embedded tissues were then stained with hematoxylin and eosin stain [59] . After staining, we microscopically examined the stained sections for the evaluation of inflammatory infiltrate. Endotoxin shock For LPS challenge, mice received intraperitoneal injections of LPS (2.5 or 5 mg kg −1 body weight). Sera were collected 2 h and 6 h after LPS challenge to test TNF-α and IL-12 productions by CBA (BD Pharmingen). Aspartate aminotransferase and alanine aminotransferase in the sera after LPS treatment for 6 and 12 h were assayed in Beijing North Institute of Biological Technology. Liver and kidney samples were fixed with formaldehyde and microscopically examined for inflammatory infiltration. Quantitative PCR analysis The inflammatory response of macrophages were induced by LPS (100 ng ml −1 ) for 6 h. The M2 macrophages were induced by IL-4 (1,000 U ml −1 ) treatment for 48 h. Total RNA was isolated with TRIzol (Invitrogen, Carlsbad, CA) and reverse transcription was performed with M-MLV superscript reverse transcriptase according to the manufacturer's instructions. Real-time PCR was performed using multiple kits (SYBR Premix Ex TaqTM, DRR041A, Takara Bio) on CFX96 (Bio-Rad). The primers used in the present study are listed in Table 2 . To determine the relative induction of cytokine mRNA in response to various stimuli, the mRNA expression levels of each gene were normalized to the expression level of the housekeeping gene hypoxanthine phosphoribosyl transferase. Table 2 Primers used for qRT–PCR analysis. Full size table Western blot assay Macrophages or MEF cells were cultured in DMEM medium with 10% FCS in 6-well plates. Cells were treated with IL-4 (100 nM) or LPS (100 ng ml −1 ) for the indicated time. After stimulation, cells were washed once in cold PBS, lysed in RIPA buffer (50 mM Tris–HCl pH 7.4, 1% NP-40, 0.25% Na-deoxycholate, 150 mM NaCl, 1 mM EDTA pH 7.4) with protease and phosphatase inhibitor cocktails (Sigma) for 10 min on a rocker at 4 °C. Protein concentration was determined using a BCA assay. Proteins samples were analysed on SDS polyacrylamide gel electrophoresis (SDS–PAGE) and transferred onto PVDF membranes (Millipore, CA) [60] . Each polyvinylidene fluoride membrane was blocked with TBST (100 mM Tris–HCl pH 7.5, 150 mM NaCl, 0.05% Tween20) with 5% non-fat dried milk for 1 h, then incubated with primary antibodies overnight on a shaker at 4 °C. The appropriate HRP-coupled secondary antibody was then added, and was detected through chemiluminescence (Millipore). Actin was used as a protein loading control. Ras GTPase pull-down assays RBD domain of Raf1 was cloned and inserted into pGEX-4t-2 vector digested with EcoRI and XhoI sites. Raf1-RBD protein was induced by 0.5 mM isopropyl-β- D -thiogalactopyranoside at 25 °C overnight in BL21 (DE3). GST-Raf1-RBD protein was purified from bacterial extracts by incubation with glutathione sepharose beads according to its manual (GE Corporate). Purity was confirmed using SDS–PAGE and Coomassie blue staining. MEF cells (kindly offered by Dr Hongbing Zhang) and bone marrow-derived macrophages were treated with LPS for 1 h, and immediately lysed. Approximately 1 mg equal amounts of the resulting supernatant fractions were incubated with GST-Raf1-RBD-agarose (containing 50 μg GST-RBD protein, which binds Ras GTPase) for 2 h and shaken at 4 °C, followed by washing the beads three times with lysis buffer. Proteins that bound to the beads were eluted in protein loading buffer and subjected to western blot analysis using antibody specific to Ras GTPase. Measurements of TSC2 GAP activity towards Ras GTPase GST-Raf1-RBD protein was prepared and purified as described above. His-Ras expressed from pET28a-Ras was purified from E. coli BL21 (DE3) cells after induction with 0.5 mM isopropyl-β- D -thiogalactopyranoside at 25 °C overnight. Bacterial lysates were prepared by freezing and thawing bacterial pellets in 1 per 50 volume PBS plus protease inhibitors followed by sonication for 15 min on ice. The His-Ras fusion protein was then purified by Ni 2+ -NTA resin (Millipore) according to the manufacturer’s instructions. Lipofectamine 2000 reagent (Invitrogen) was used for transfecting 293T cells with p3XFlag-TSC2Δ400 in 10 cm culture dishes. Twenty four hours after transfection, cells were treated with Flag lysis ((50 mM Tris–HCl, pH 7.4, 150 mM NaCl, 1 mM EDTA, 1% Triton X-100) plus protease inhibitors. Flag-tagged proteins were then immunoprecipitated and purified with 50 μl M2-agarose affinity gel slurry (Sigma-Aldrich) according to the user manual. The Eluted His-Ras, GST-Raf1-RBD and Flag-TSC2Δ400 were then analysed and quantitated by SDS–PAGE. His-Ras (5 μg) was loaded with 2 μl 100 mM GTP by incubation on ice in 100 μl GTP-loading buffer (50 mM HEPES pH 7.5, 1 mM EDTA and 0.1 mg ml −1 bovine serum albumin plus protease inhibitors). After 30 min, 2.5 μl 1 M MgCl 2 and 20 μl 10 mM GDP were added, mixed and separated into four aliquots. GAP assays were initiated by the addition of 500 ng Flag-TSC2Δ400 protein to each aliquot. Assays were performed at room temperature with constant agitation for 0, 5, 10 or 20 min. Reactions were stopped by the addition of 500 μl wash buffer (50 mM HEPES pH 7.5, 0.5 M NaCl, 0.1% Triton X-100, 5 mM MgCl 2 , 0.005% SDS plus protease inhibitors). M2-agarose was removed and active Ras GTPase was then immunoprecipitated with 50 μg GST-Raf1-RBD for 2 h. The quantity of active Ras GTPase was determined by western blots. Overexpression of C/EBPβ in bone marrow-derived macrophages An adenoviral construct encoding C/EBPβ was prepared with a ViraPower adenovirus expression system (Invitrogen) according to the manufacturer’s instructions and previous reports [61] . Briefly, cDNA that encodes for the C/EBPβ gene and Ubic promoter-GFP fragment were subcloned into the pENTR vector. As a control, only Ubic promoter-GFP fragment was subcloned into the pENTR vector. These constructs were then recombined with pAd/CMV/V5-DEST, using LR Clonase II (Invitrogen), according to the manufacturer’s protocol, to generate the pAd plasmids. The plasmids were linearized using PacI and then transfected into 293A cells with Lipofectamine 2000. After 10 days, cells from wells showing 100% cytopathic effect were collected by scraping, lysed with three rounds of freeze/thaw and centrifuged to collect the supernatant. One more round of infection with the supernatant was performed to enhance the viral titre. The viral titres were determined by plaque-forming assays with 293A cells. Bone marrow-derived macrophages were prepared as described above and infected with the freshly prepared viral supernatant (50% viral supernatant containing empty vector or CEBPβ, supplied with 50% DMEM complete media) for 24 h. The cells were then washed and stimulated with IL-4 (1,000 U ml −1 ) for additional 48 h. Statistical analysis All data are presented as the mean±s.d. Two-way ANOVA analysis was used for comparison among multiple groups with SPSS 16.0 software. Student’s unpaired t -test for comparison of means was used to compare between two groups. Log-rank tests were used for mouse survival assays. A P value less than 0.05 was considered to be statistically significant. How to cite this article : Zhu, L. et al. TSC1 controls macrophage polarization to prevent inflammatory disease. Nat. Commun. 5:4696 doi: 10.1038/ncomms5696 (2014).